FAK-heterozygous mice display enhanced tumour angiogenesis Genetic ablation of endothelial focal adhesion kinase (FAK) can inhibit pathological angiogenesis, suggesting that loss of endothelial FAK is sufficient to reduce neovascularization. Here we show that reduced stromal FAK expression in FAK-heterozygous mice unexpectedly enhances both B16F0 and CMT19T tumour growth and angiogenesis. We further demonstrate that cell proliferation and microvessel sprouting, but not migration, are increased in serum-stimulated FAK-heterozygous endothelial cells. FAK-heterozygous endothelial cells display an imbalance in FAK phosphorylation at pY397 and pY861 without changes in Pyk2 or Erk1/2 activity. By contrast, serum-stimulated phosphorylation of Akt is enhanced in FAK-heterozygous endothelial cells and these cells are more sensitive to Akt inhibition. Additionally, low doses of a pharmacological FAK inhibitor, although too low to affect FAK autophosphorylation in vitro , can enhance angiogenesis ex vivo and tumour growth in vivo . Our results highlight a potential novel role for FAK as a nonlinear, dose-dependent regulator of angiogenesis where heterozygous levels of FAK enhance angiogenesis. The non-receptor tyrosine kinase, focal adhesion kinase (FAK), can signal downstream of integrins and growth factor receptors [1] . FAK is expressed ubiquitously and has essential roles in a number of cellular processes, including proliferation and migration, which are important angiogenic processes. FAK is autophosphorylated at Y397 following integrin activation and additionally this site acts to recruit members of the Src-family kinases [2] , [3] , [4] . The proximity of Src-family kinases to FAK is thought to result in its phosphorylation at other sites, including Y861, and this may cause activation of downstream effectors including Erk and Akt [5] , [6] . Previous reports have highlighted that the kinase activity, and phosphorylation of FAK at Y397 and Y861, are important regulators of angiogenic responses in vitro [3] , [7] , [8] , [9] . Nonetheless, how the activity of these sites affect the tumour stromal influence on tumorigenesis has never been addressed. Genetic studies also have indicated a role for FAK in angiogenesis in vivo . For example, the global deletion of FAK results in an early embryonic lethal phenotype with defects in the vascular system [10] . Constitutive FAK-deletion specifically in vascular endothelial cells (ECs) caused embryos to die between E10.5 and E13.5, which coincides with the onset of embryonic vascular system development [11] , [12] , while overexpression of FAK in ECs has led to enhanced blood vessel density during various angiogenic processes [13] . Although one report suggests that the inducible deletion of endothelial FAK in End-SCL-Cre ERT adult mice failed to affect adult angiogenesis, this apparently was because of induced compensation by a related family member, Pyk2 (ref. 14 ). We have shown previously that endothelial-specific loss of FAK in Pdgfb-iCreER T2 ;FAK fl/fl mice inhibit tumour angiogenesis [15] . Together, these data suggest that loss of FAK can be sufficient to inhibit pathological angiogenesis. Conversely, although FAK-knockdown inhibited cell migration and tube formation in vitro [10] , others have shown that FAK-phosphorylation [16] and levels of expression are decreased during the early stage of an in vitro model of angiogenesis [17] . Such, apparently contradicting results suggest that FAK may have nonlinear dose-dependent roles in angiogenesis with varied FAK levels differentially affecting angiogenesis. Indeed, the embryonic development of FAK-heterozygous mice is severely retarded, but these defects are overcome by birth and FAK-heterozygous mice are born at normal Mendelian ratios with no gross abnormalities [18] . In addition, although FAK is expressed ubiquitously, its expression and activity levels can vary between cells and even within the same cell type [4] , [19] , suggesting that examining the effects of partial loss of endothelial FAK may provide us with more physiologically relevant information about its roles in vivo . Here, we have tested the influence that subtle changes in stromal-FAK levels may have on tumour growth and angiogenesis, by utilizing FAK-heterozygous mice [20] . FAK-heterozygous mice display half the normal levels of FAK protein. We show that FAK-heterozygous mice exhibit: (1) enhanced B16F0 melanoma and CMT19T lung carcinoma tumour growth, (2) increased formation of perfused tumour blood vessels and (3) elevated neovascularization in vivo . At the molecular level, we have determined that the ratio of FAK phosphorylation at Y861:Y397 is misbalanced and that the relative phosphorylation of Akt is elevated in FAK-heterozygous ECs. In agreement with this, FAK-heterozygous ECs exhibit increased sensitivity to Akt inhibition. Lastly, low doses of the FAK inhibitor, PF573228, can phenocopy the responses in FAK-heterozygotes. Taken together, these data suggest that FAK has a nonlinear dose-dependent effect in angiogenesis with partial loss of FAK function being sufficient to enhance pathological angiogenic responses. Tumour growth and angiogenesis in FAK-heterozygous mice Tumour growth has been associated with enhanced tumour cell FAK expression, but the role of stromal-FAK is less well understood. Although some data indicate that total loss of FAK can inhibit angiogenic processes [10] , [11] , [12] , [15] , others suggest that it may have a nonlinear dose-dependent role in neovascularizing events [4] , [16] , [17] , [19] . Using FAK-heterozygous mice [20] we investigated the effect of partial loss of stromal FAK on tumour growth and angiogenesis. These mice carry only one FAK allele and western blot analysis confirmed that FAK protein expression was reduced to 50% in FAK-heterozygous tissues when compared with wild-type ( Supplementary Fig. S1 ). To assess whether decreased FAK levels have a role in tumour growth, we injected syngeneic B16F0 melanoma cells or CMT19T lung carcinoma cells into the flanks of age- and sex-matched FAK-heterozygous mice and wild-type littermates. Two weeks post inoculation, both B16F0 and the CMT19T tumours from FAK-heterozygous animals were significantly larger than those from wild-type controls ( Fig. 1a ). Indeed, tumour growth was increased significantly in FAK-heterozygous mice when compared with wild-type controls over time ( Supplementary Fig. S2 ). These data indicate that partial loss of FAK in the tumour stroma is sufficient to enhance tumour growth. 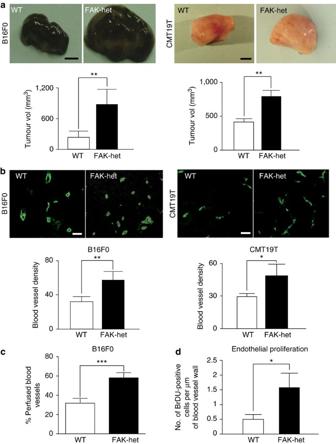Figure 1: Increased tumour size and angiogenesis in FAK-heterozygous mice. (a) Subcutaneous 14-day-old B16F0 and CMT19T tumour sizes were elevated significantly in FAK-heterozygous (FAK-het) mice when compared with similar tumours in age- and sex-matched wild-type (WT) control littermates.Top panels, representative images of macroscopic appearance of tumours. Bar charts represent mean tumour volumes, +s.e.m;n=20 mice per genotype for the CMTs studies andn=30 mice per genotype for the B16F0 studies, Mann–Whitney rank-sum test,**P<0.01. (b) Endomucin staining patterns of midline sections of age-matched, size-matched B16F0 and CMT19T tumours from WT and FAK-het mice. Microvessel density is given as the number of blood vessels per mm2of midline tumour section. Microvessel density in B16F0 and CMT19T tumours was significantly greater in FAK-het mice when compared with WT controls. Bar charts represent mean tumour blood vessel density of age-matched, size-matched tumours+s.e.m.n=20 CMTs tumours andn=30 B16F0 tumours per genotype, Student’st-test,**P<0.01,*P<0.06. (c) The number of functional tumour blood vessels was assessed by intravenous injection of PE-PECAM antibody before tumour excision in FAK-het and WT control mice. B16F0 tumours grown in FAK-het mice had an increased number of functional tumour blood vessels compared with WT littermates. Bar chart represents the percentage of perfused vessels over total blood vessels per midline tumour section from WT and FAK-het mice+s.e.m.n=10 tumours per genotype, Student’st-test, ***P<0.001. (d) Tumour endothelial proliferation was enhanced in FAK-het mice. Bar chart represents mean number of BrdU-positive ECs per blood vessel perimeter length (μm) in midline B16F0 tumour sections from WT and FAK-het mice+s.e.m.n=5 tumours per genotype, Student’st-test,*P<0.04. Scale bars, 0.3 cm (a), 30 μm (b). Figure 1: Increased tumour size and angiogenesis in FAK-heterozygous mice. ( a ) Subcutaneous 14-day-old B16F0 and CMT19T tumour sizes were elevated significantly in FAK-heterozygous (FAK-het) mice when compared with similar tumours in age- and sex-matched wild-type (WT) control littermates. Top panels , representative images of macroscopic appearance of tumours. Bar charts represent mean tumour volumes, +s.e.m; n =20 mice per genotype for the CMTs studies and n =30 mice per genotype for the B16F0 studies, Mann–Whitney rank-sum test, **P <0.01. ( b ) Endomucin staining patterns of midline sections of age-matched, size-matched B16F0 and CMT19T tumours from WT and FAK-het mice. Microvessel density is given as the number of blood vessels per mm 2 of midline tumour section. Microvessel density in B16F0 and CMT19T tumours was significantly greater in FAK-het mice when compared with WT controls. Bar charts represent mean tumour blood vessel density of age-matched, size-matched tumours+s.e.m. n =20 CMTs tumours and n =30 B16F0 tumours per genotype, Student’s t -test, **P <0.01, *P <0.06. ( c ) The number of functional tumour blood vessels was assessed by intravenous injection of PE-PECAM antibody before tumour excision in FAK-het and WT control mice. B16F0 tumours grown in FAK-het mice had an increased number of functional tumour blood vessels compared with WT littermates. Bar chart represents the percentage of perfused vessels over total blood vessels per midline tumour section from WT and FAK-het mice+s.e.m. n =10 tumours per genotype, Student’s t -test, *** P <0.001. ( d ) Tumour endothelial proliferation was enhanced in FAK-het mice. Bar chart represents mean number of BrdU-positive ECs per blood vessel perimeter length (μm) in midline B16F0 tumour sections from WT and FAK-het mice+s.e.m. n =5 tumours per genotype, Student’s t -test, *P <0.04. Scale bars, 0.3 cm ( a ), 30 μm ( b ). Full size image To examine whether the elevated tumour size in FAK-heterozygous mice correlated with any change in tumour angiogenesis midline sections of size-matched, age-matched tumours were analysed. Double immunostaining for platelet endothelial cell adhesion molecule (PECAM) and FAK, revealed that endothelial FAK levels were decreased significantly in tumour blood vessels in FAK-heterozygous mice when compared with wild-type controls and that the levels varied widely in the wild-type mice ( Supplementary Fig. S3 ). In contrast, FAK levels were indistinguishable in the tumour cell compartment between both genotypes, suggesting that stromal FAK did not affect tumour cell FAK levels ( Supplementary Fig. S4 ). Tumour blood vessel density was defined by counting the total number of blood vessels across entire midline sections and dividing by the tumour section area. Results revealed that blood vessel density was increased in both B16F0 and CMT19T tumours grown in FAK-heterozygous mice when compared with control mice ( Fig. 1b ). Furthermore, the number of functional, PE-PECAM antibody perfused, blood vessels was also increased in B16F0 tumours grown in FAK-heterozygous mice ( Fig. 1c ). Enhanced tumour blood vessel perfusion has been associated with increased tumour growth previously [21] , [22] . These data correlated with a significant increase in the number of BrdU-positive vessels in B16F0 tumours from FAK-heterozygous mice when compared with those from control mice ( Fig. 1d ). Importantly, the blood vessel density in unchallenged skin was not changed between genotypes, suggesting that the enhanced tumour angiogenesis was not due to elevated blood vessel numbers in untreated FAK-heterozygous mice ( Supplementary Fig. S5 ). Taken together, these data point towards a role for stromal FAK in the regulation of angiogenesis. Angiogenesis can be affected by various cell types other than ECs. For example, the formation of stable angiogenic vessels is associated with the recruitment of pericytes. Our data showed that the number of tumour blood vessels associated with α-smooth muscle actin-positive pericytes was similar between the two genotypes, suggesting that vessel maturation was not affected by FAK heterozygosity ( Supplementary Fig. S6 ). Any changes in tumour vascularity did not appear to correlate with changes in tumour hypoxia, apoptosis or levels of serum vascular endothelial growth factor (VEGF) between the two genotypes ( Supplementary Figs. S7, S8 and S9 ). Although, changes in inflammatory cell infiltrate have been reported to enhance neovascularization [23] , [24] no significant differences in the relative level of macrophage (Gr1+ or F4/80+) or leukocyte (CD45+) infiltration was observed between tumours from FAK-heterozygous or control animals ( Supplementary Fig. S10 ). Overall, although we cannot rule out a non-cell autonomous affect on the enhanced angiogenesis observed in FAK-heterozygous mice, we have no evidence for changes in any of the cell types tested other than in ECs. VEGF is a major pro-angiogenic growth factor. To determine whether the changes observed during tumour angiogenesis could be seen in a tumour-free environment, VEGF impregnated sponges were implanted subcutaneously into FAK-heterozygous and wild-type mice to stimulate blood vessel growth. Results showed that FAK-heterozygous mice had a higher infiltration of blood vessels into sponges with or without VEGF when compared with similarly treated wild-type controls ( Fig. 2 ). Indeed, there was no difference in the fold-increase of in vivo blood vessel infiltration in wild-type mice when compared with FAK-heterozygous mice, suggesting that the enhanced angiogenic response was not VEGF-specific. Thus, our data suggested that in vivo VEGF-mediated responses were not enhanced in FAK-heterozygous mice per se . This notion was corroborated by western blot analysis for VEGF-receptor 2 protein expression and downstream signalling activity in purified ECs. Our results showed that although FAK-heterozygous ECs displayed approximately half the levels of total FAK, as expected, there was no change in VEGF-stimulated levels of VEGF-receptor 2, phospho-VEGF-receptor 2 or downstream effectors such as p130Cas, phospho-p130Cas, total Erk1/2 or phospho-Erk1/2. In short, our data indicated that partial loss of FAK in FAK-heterozygous ECs does not affect VEGF-mediated signalling specifically ( Supplementary Fig. S11 ). In addition, VEGF-stimulation did not affect the migration speed of FAK-heterozygous cells ( Supplementary Fig. S12 ). Therefore, although beyond the scope of the present study, other angiogenic factors may have a role in triggering the enhanced angiogenic response in FAK-heterozygous mice. Thus we focused on the effect of partial loss of FAK on serum-stimulated endothelial activity. 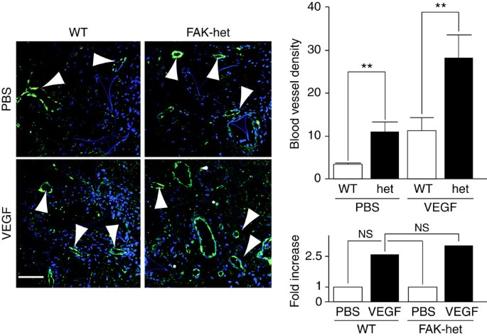Figure 2: Tumour-free angiogenesis is enhanced in FAK-heterozygous mice. Sponges implanted into the flanks of either FAK-het mice or WT controls were injected with VEGF or PBS every 2 days for 2 weeks. At 2 weeks post implantation,in vivoangiogenesis was assessed by counting the numbers of blood vessels per mm2in sponge sections from WT and FAK-het mice. VEGF-treatment enhanced angiogenesis in both WT and FAK-het mice. However, quantitation showed that angiogenesis is elevated both at the baseline level, PBS-treated and after VEGF-stimulation (VEGF) in FAK-het mice. Upper bar chart represents mean numbers of blood vessels per mm2of sponge section+s.e.m. Lower bar chart shows that the relative fold-increase in microvessel density of FAK-het mice over WT controls was similar for both PBS and VEGF-treated sponges. Arrowheads indicate blood vessels. 4',6-Diamidino-2-phenylindole-stained nuclei, blue,n=7 WT andn=10 FAK-het mice, Student’st-test, NS, no statistically significant difference, **P<0.05. Scale bar, 100 μm. Figure 2: Tumour-free angiogenesis is enhanced in FAK-heterozygous mice. Sponges implanted into the flanks of either FAK-het mice or WT controls were injected with VEGF or PBS every 2 days for 2 weeks. At 2 weeks post implantation, in vivo angiogenesis was assessed by counting the numbers of blood vessels per mm 2 in sponge sections from WT and FAK-het mice. VEGF-treatment enhanced angiogenesis in both WT and FAK-het mice. However, quantitation showed that angiogenesis is elevated both at the baseline level, PBS-treated and after VEGF-stimulation (VEGF) in FAK-het mice. Upper bar chart represents mean numbers of blood vessels per mm 2 of sponge section+s.e.m. Lower bar chart shows that the relative fold-increase in microvessel density of FAK-het mice over WT controls was similar for both PBS and VEGF-treated sponges. Arrowheads indicate blood vessels. 4',6-Diamidino-2-phenylindole-stained nuclei, blue, n =7 WT and n =10 FAK-het mice, Student’s t -test, NS, no statistically significant difference, ** P <0.05. Scale bar, 100 μm. Full size image FAK heterozygosity enhances cell survival and tube formation In order to determine the cellular mechanisms underlying the enhanced pathological angiogenesis observed in FAK-heterozygous mice, ECs from FAK-heterozygous and control mice were isolated and subjected to a number of cellular assays. As an indication of relative survival, ECs grown in full growth medium were assayed; for (4-[3-(4-Iodophenyl)-2-(4-nitrophenyl)-2H-5-tetrazolio]-1,3-benzene disulfonate (WST-1) metabolism. Interestingly, FAK-heterozygous ECs demonstrated significantly increased WST-1 metabolism when compared with control cells ( Fig. 3a ), suggesting that partial loss of FAK enhances endothelial survival. In contrast, using Dunn chamber assays to determine the effect of partial FAK loss on cell migration, no statistically significant differences in serum-mediated migration speed or persistence of cell migration were observed between genotypes ( Fig. 3b ). 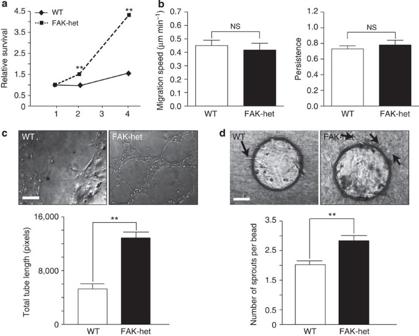Figure 3: Characterization of endothelial cells isolated from FAK-heterozygous mice. (a) Using the WST-1 assay, primary EC survivalin vitrowas assessed. Graph shows that, over 4 days, survival of FAK-heterozygous (FAK-het) ECs was enhanced significantly over wild-type (WT) EC survival,n=44 wells per condition, 2,500 cells per well, Student’st-test,**P<0.001. (b) Serum-stimulated speed of cell migration and persistence was assessed in Dunn chambers for WT and FAK-het ECs. No difference in speed or persistence was detected. Values are given as means+s.e.m.n=57 WT andn=62 FAK-het cells, Student’st-test, NS, no statistically significant difference. (c) Two-dimensional tube formation (total tube length) of FAK-het ECs was enhanced significantly when compared with WT cells. Upper panels, representative images of endothelial tubes formed by WT and FAK-het primary ECs on Matrigel,n=3, Student’st-test,**P<0.01. (d) Three-dimensional tube formation of FAK-het ECs was elevated significantly when compared with WT ECs. Representative images of endothelial sprouts from beads coated with WT and FAK-het cells cultured on beads in fibroblast-containing fibrin gel. Bar chart represents mean number of endothelial sprouts per bead+s.e.m., for WT and FAK-het ECs cultured on beads in fibroblast-containing fibrin gel. Arrows indicate endothelial sprouts,n=54 WT andn=103 FAK-het beads, three independent experiments, Student’st-test,***P<0.0005. Scale bars incandd, 50 μm. Figure 3: Characterization of endothelial cells isolated from FAK-heterozygous mice. ( a ) Using the WST-1 assay, primary EC survival in vitro was assessed. Graph shows that, over 4 days, survival of FAK-heterozygous (FAK-het) ECs was enhanced significantly over wild-type (WT) EC survival, n =44 wells per condition, 2,500 cells per well, Student’s t -test, **P <0.001. ( b ) Serum-stimulated speed of cell migration and persistence was assessed in Dunn chambers for WT and FAK-het ECs. No difference in speed or persistence was detected. Values are given as means+s.e.m. n =57 WT and n =62 FAK-het cells, Student’s t -test, NS, no statistically significant difference. ( c ) Two-dimensional tube formation (total tube length) of FAK-het ECs was enhanced significantly when compared with WT cells. Upper panels, representative images of endothelial tubes formed by WT and FAK-het primary ECs on Matrigel, n =3, Student’s t -test, **P <0.01. ( d ) Three-dimensional tube formation of FAK-het ECs was elevated significantly when compared with WT ECs. Representative images of endothelial sprouts from beads coated with WT and FAK-het cells cultured on beads in fibroblast-containing fibrin gel. Bar chart represents mean number of endothelial sprouts per bead+s.e.m., for WT and FAK-het ECs cultured on beads in fibroblast-containing fibrin gel. Arrows indicate endothelial sprouts, n =54 WT and n =103 FAK-het beads, three independent experiments, Student’s t -test, ***P <0.0005. Scale bars in c and d , 50 μm. Full size image Tube formation is a vital step of angiogenesis. ECs are known to form tubular structures when grown on a two-dimensional Matrigel substrate [25] . FAK-heterozygous cells spontaneously formed more tubular structures than wild-type control cells in two-dimensional Matrigel assays ( Fig. 3c ). In addition, in three-dimensional tubulogenesis assays, FAK-heterozygous ECs cultured on fibrinogen-coated beads, in the presence of full endothelial growth medium and a fibroblast feeder layer, developed significantly higher numbers of tubular sprouts than wild-type cells grown under similar conditions ( Fig. 3d ). In short, the partial loss of FAK in ECs confers a spontaneous ability to enhance angiogenic responses that is independent of effects on EC migration. Pyk2 does not compensate FAK heterozygosity Changes in FAK activity have been correlated with changes in its levels of phosphorylation [3] . In addition, apart from FAK, a related family member, Pyk2 has also been reported to be expressed in ECs and has, in some circumstances, been implicated in compensating for FAK [14] . We next explored the expression and phosphorylation levels of FAK and Pyk2 in FAK-heterozygous and wild-type ECs. Immunofluorescence analysis of total FAK, pY397-FAK and pY861-FAK showed that, although the intensity levels of total FAK and pY397-FAK were decreased in the FAK-heterozygous cells ( Fig. 4a ), the level of FAK-phosphorylation, specifically at Y861, was similar in FAK-heterozygous and wild-type ECs ( Fig. 4a ). Furthermore, western blot analysis of wild-type and FAK-heterozygous EC extracts confirmed that FAK levels were reduced in FAK-heterozygous ECs, and revealed a correlation with a decrease in pY397-FAK, but not pY861-FAK levels ( Fig. 4b ). Consequently, although the ratio of pY397-FAK/total FAK remained the same between the two genotypes, the ratio of pY861-FAK/total FAK displayed a twofold increase in FAK-heterozygous cells when compared with wild-type ECs. Moreover, a reduction of FAK levels in ECs did not cause any changes in the expression or phosphorylation of Pyk2 ( Fig. 4b ). FAK is also known to have an important role in the dynamic regulation of focal contacts and the organization of the actin cytoskeleton [2] . Our data revealed that FAK heterozygosity was not sufficient to alter the organization of endothelial F-actin bundles ( Fig. 5a ). In addition, immunofluorescence and western blot studies suggested that paxillin, talin and vinculin levels were unchanged between genotypes ( Fig. 5a ). Taken together, FAK heterozygosity does not appear to result in overt compensatory mechanisms involving Pyk2 or other focal contact proteins. 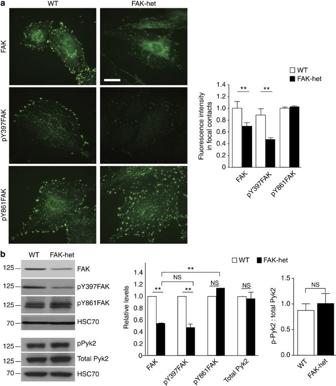Figure 4: Imbalance between pFAK-Y397 and pFAK-Y861 in FAK-heterozygous cells. (a) Immunocytochemistry for FAK, pY397-FAK and pY861-FAK in cultured wild-type (WT) and FAK-heterozygous (FAK-het) ECs. Results show that the expression of FAK and pY397-FAK were reduced in FAK-het cells but that the expression of pY861-FAK was unchanged. Bar chart represents mean relative fluorescence signal intensity of FAK, pY397-FAK and pY861-FAK in FAK-het, and WT ECsin vitro+s.e.m.n=5, Student’st-test, **P<0.01. (b) Western blot analysis of FAK, pY397-FAK, pY861-FAK, Pyk2 and phosphorylated Pyk2 (pPyk2) in cultured WT and FAK-het ECs lysates. HSC70 acted as a loading control. Results show that expression levels of total FAK and pY397-FAK are similarly reduced in FAK-het cells but that pY861-FAK levels are unchanged between genotypes, resulting in significantly elevated ratio of pY861-FAK/total FAK while the ratio of pY397-FAK/total FAK remains the same in FAK-het ECs. The expression of Pyk2 and the ratio of pPyk2: total-Pyk2 are similar in FAK-het and WT ECs. Bar chart represents densitometric readings relative to WT+s.e.m.n=3 independent experiments, Student’st-test**P<0.01, NS, no statistically significant difference. Scale bar ina, 25 μm. Figure 4: Imbalance between pFAK-Y397 and pFAK-Y861 in FAK-heterozygous cells. ( a ) Immunocytochemistry for FAK, pY397-FAK and pY861-FAK in cultured wild-type (WT) and FAK-heterozygous (FAK-het) ECs. Results show that the expression of FAK and pY397-FAK were reduced in FAK-het cells but that the expression of pY861-FAK was unchanged. Bar chart represents mean relative fluorescence signal intensity of FAK, pY397-FAK and pY861-FAK in FAK-het, and WT ECs in vitro +s.e.m. n =5, Student’s t -test, ** P <0.01. ( b ) Western blot analysis of FAK, pY397-FAK, pY861-FAK, Pyk2 and phosphorylated Pyk2 (pPyk2) in cultured WT and FAK-het ECs lysates. HSC70 acted as a loading control. Results show that expression levels of total FAK and pY397-FAK are similarly reduced in FAK-het cells but that pY861-FAK levels are unchanged between genotypes, resulting in significantly elevated ratio of pY861-FAK/total FAK while the ratio of pY397-FAK/total FAK remains the same in FAK-het ECs. The expression of Pyk2 and the ratio of pPyk2: total-Pyk2 are similar in FAK-het and WT ECs. Bar chart represents densitometric readings relative to WT+s.e.m. n =3 independent experiments, Student’s t -test **P <0.01, NS, no statistically significant difference. Scale bar in a , 25 μm. 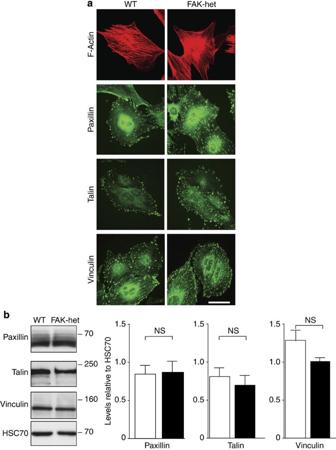Figure 5: Expression of focal contact proteins in FAK-heterozygous endothelial cells. (a) Immunocytochemistry for F-actin, paxillin, talin and vinculin in cultured wild-type (WT) and FAK-heterozygous (FAK-het) ECs. (b) Western blot analysis of paxillin, talin and vinculin in cultured WT and FAK-het EC lysates. HSC70 acted as a loading control. Results show that overall expression levels of paxillin, talin and vinculin are unchanged between genotypes. Bar chart represents densitometric readings+s.e.m.n=4 independent experiments, Student’st-test, NS, no statistically significant difference. Scale bar ina, 25 μm. Full size image Figure 5: Expression of focal contact proteins in FAK-heterozygous endothelial cells. ( a ) Immunocytochemistry for F-actin, paxillin, talin and vinculin in cultured wild-type (WT) and FAK-heterozygous (FAK-het) ECs. ( b ) Western blot analysis of paxillin, talin and vinculin in cultured WT and FAK-het EC lysates. HSC70 acted as a loading control. Results show that overall expression levels of paxillin, talin and vinculin are unchanged between genotypes. Bar chart represents densitometric readings+s.e.m. n =4 independent experiments, Student’s t -test, NS, no statistically significant difference. Scale bar in a , 25 μm. Full size image Effect of FAK heterozygosity on Akt signalling FAK can affect both integrin and growth factor signalling by regulating downstream targets, such as Erk1/2 and Akt [1] , [3] , [6] , [8] . Our results show that serum-stimulated phosphorylation of Erk1/2 was not significantly altered in FAK-heterozygous ECs when compared with wild-type controls. In contrast, although the absolute expression levels of pAkt did not appear to change between genotypes ( Fig. 6a ), the levels of total Akt were reduced significantly in FAK-heterozygous ECs compared with wild-type ECs ( Supplementary Fig. S13 ). This resulted in a significant increase in the ratio of pAkt/ total Akt in FAK-heterozygous ECs when compared with wild-type controls ( Fig. 6a ). To establish whether this increase in pAkt/ total Akt ratio was functionally linked to the increased angiogenic activity of FAK-heterozygotes, we tested the affect of Akt inhibition on angiogenic responses ex vivo . FAK-heterozygous and wild-type aortic rings were treated with the Akt inhibitor VIII, which selectively inhibits the kinase activity of Akt1/2. High doses (10 μM range) of the Akt VIII inhibitor were able to inhibit microvessel sprouting in both FAK-heterozygous and wild-type aortic rings. However, the enhanced Akt-sensitivity of FAK-heterozygotes was illustrated by their decreased sprouting response to lower doses (1 μM range) of the Akt inhibitor that did not affect wild-type aortic rings ( Fig. 6b ). These data suggest that the elevated Akt activation could contribute to the pro-angiogenic phenotype of FAK-heterozygous mice. 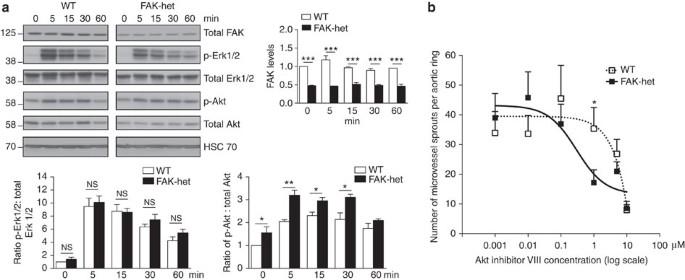Figure 6: Effect of FAK heterozygosity on Akt signalling. (a) Western blot analysis of total FAK, phosphorylated-Erk1/2, total Erk1/2, phosphorylated-Akt and total Akt, in cultured wild-type (WT) and FAK-heterozygous (FAK-het) EC lysates after serum-stimulation for 0, 5, 15, 30 and 60 min. HSC70 acted as loading control. Bar charts show mean densitometric readings of total FAK levels; ratios of p-Erk1/2:total Erk1/2; and ratios of pAkt:total Akt from WT and FAK-het EC lysates after serum-stimulation for 0, 5, 15, 30 and 60 min,+s.e.m.n=5 (FAK),n=3 (Erk) andn=4 (Akt) independent experiments, Student’st-test, ***P<0.001, **P<0.01, *P<0.05, NS, no statistically significant difference. (b) Microvessel sprouting of FAK-het aortic rings displays higher sensitivity to inhibition of Akt activity than WT controls with lower dose of Akt inhibitor causing a reduction in microvessel sprouting without affecting wild-type aortic rings. Bar chart represents the fitting curves of the average number of microvessel aortic sprouts+s.e.m. relative to the log concentrations of Akt inhibitor VIII,n= 12 aortic rings per treatment, Student’st-test, *P<0.05. Figure 6: Effect of FAK heterozygosity on Akt signalling. ( a ) Western blot analysis of total FAK, phosphorylated-Erk1/2, total Erk1/2, phosphorylated-Akt and total Akt, in cultured wild-type (WT) and FAK-heterozygous (FAK-het) EC lysates after serum-stimulation for 0, 5, 15, 30 and 60 min. HSC70 acted as loading control. Bar charts show mean densitometric readings of total FAK levels; ratios of p-Erk1/2:total Erk1/2; and ratios of pAkt:total Akt from WT and FAK-het EC lysates after serum-stimulation for 0, 5, 15, 30 and 60 min,+s.e.m. n =5 (FAK), n =3 (Erk) and n =4 (Akt) independent experiments, Student’s t -test, *** P <0.001 , **P <0.01 , *P <0.05, NS, no statistically significant difference. ( b ) Microvessel sprouting of FAK-het aortic rings displays higher sensitivity to inhibition of Akt activity than WT controls with lower dose of Akt inhibitor causing a reduction in microvessel sprouting without affecting wild-type aortic rings. Bar chart represents the fitting curves of the average number of microvessel aortic sprouts+s.e.m. relative to the log concentrations of Akt inhibitor VIII, n = 12 aortic rings per treatment, Student’s t -test, * P <0.05. Full size image Low-dose FAK inhibition increases tumour growth and angiogenesis To determine whether inhibition of FAK can enhance microvessel sprouting, we tested the effect of treatment with various concentrations of FAK inhibitor PF573228 (ref. 26 ) in ex vivo aortic ring assays. Interestingly, although high concentrations (1 μM) of PF573228 reduced microvessel sprouting from aortic rings, low concentrations (0.01 μM) of the inhibitor enhanced the numbers of microvessel sprouts significantly ( Supplementary Fig. S14 ), phenocopying the enhanced angiogenic activity observed in FAK-heterozygous mice. PF573228 has not been reported to have been used previously in in vivo experiments. However, the related PF-562271 FAK inhibitor, which display similar inhibitory activity in in vitro functional assays [26] , [27] , [28] , has been shown to inhibit tumour growth in mice at 50 mg kg −1 dose (refs 27 , 28 , 29 ). Therefore, we treated wild-type mice bearing B16F0 tumours with 12.5 mg kg −1 PF573228—a suboptimal dose of this inhibitor. Tumour growth was enhanced in mice treated with 12.5 mg kg −1 PF573228 compared with placebo-treated mice ( Supplementary Fig. S15 ). Further analysis showed that tumour blood vessel density was also enhanced significantly in mice treated with 12.5 mg kg −1 PF573228 ( Supplementary Fig. S15 ). Taken together, these findings indicate that FAK can have a nonlinear dose-dependent function in regulating tumour growth and angiogenesis. Although FAK is ubiquitously expressed, its actual levels of expression can vary within tissues and even within individual cell types [4] , [19] . Indeed, here we have observed a wide range of FAK expression levels in ECs from wild-type mice. These observations lead to the question of how different levels of FAK might regulate biological outcome—a relatively unexplored field of research. Some reports have suggested that an increase in FAK within the whole tumour correlates with tumour progression, but in contrast high levels of FAK do not always predict outcome [3] , [29] , [30] , [31] , [32] , [33] , [34] , [35] , [36] . Given the emerging importance of the tumour stroma in regulation of cancer progression, we speculate that the influence of stromal-FAK on tumour growth may be important. Indeed with the development of FAK inhibitors as potential anticancer drugs [37] , and the fact that complete pharmacological inhibition of FAK may be difficult to maintain in vivo , elucidating the effects of different levels of stromal-FAK in cancer progression becomes a priority [38] . Our data show that stromal-FAK heterozygosity is sufficient to enhance tumour growth and tumour angiogenesis. This does not correlate with any obvious changes in endothelial expression of focal adhesion proteins or cellular migration, but does correlate with enhanced EC proliferation and relative Akt activity levels. Thus, our results establish a new role for FAK in the regulation of angiogenesis. Previous genetic ablation work has highlighted an apparent requirement for FAK during developmental and postnatal angiogenesis [10] , [11] , [12] , [15] . However, in adult organisms the total deletion of FAK is unlikely to be of physiological relevance. Thus, studying the effect of reduced levels of FAK may provide us with new information about the roles of this signalling effector. Our data suggest that heterozygous levels of FAK can elevate angiogenic responses and our results are corroborated by other reports [16] , [17] . For example, FAK-heterozygous embryos show retarded embryonic development but, by birth, appear normal [18] , suggesting that heterozygous levels of FAK might allow for some compensation that overcomes the embryonic defect. Additionally, in vitro studies have indicated that, during the first, but not latter, phases of angiogenesis, FAK levels are reduced, suggesting that FAK may have a nonlinear dose-dependent effect in angiogenic processes in vitro [16] , [17] . The tumour stroma consists of various cell types including ECs, smooth muscle cells/pericytes and inflammatory cells. It is conceivable that the enhanced angiogenic responses in FAK-heterozygous mice may be due to the upregulation of some or all of these non-EC types. However, we found no evidence for the increase in the numbers of mural cells or immune infiltrating cells in tumours grown in FAK-heterozygous mice or the number of vessels with associated pericytes. Thus, although we cannot rule out a non-cell autonomous effect, here we have focused on the endothelial compartment where we have observed FAK-dependent changes in molecular profiles and EC function. Our data demonstrate that FAK heterozygosity is sufficient to affect ECs, by increasing endothelial cell proliferation and sprout formation, but without affecting overall migration speed of these cells. Pyk2, a member of the FAK family, has been reported previously to compensate for the loss of FAK [14] . However, we did not observe any changes in Pyk2 levels or phosphorylation in the FAK-heterozygous ECs. In contrast, in FAK-heterozygous ECs, although phosphorylation of FAK at Y397 is reduced, the levels of pY861-FAK surprisingly, remain high. The ratio of pY397/ total FAK remains the same, whereas the ratio of pY861/total FAK is increased. Although it has been proposed that phosphorylation of Y397 is required for conformational changes that trigger the phosphorylation of Y861 (refs 5 , 6 , 39 ), other studies have reported enhanced phosphorylation of Y861-FAK without alterations in pY397 levels or FAK activity, suggesting that the uncoupling of these two FAK phosphorylation sites can occur [7] , [40] , [41] , [42] . In addition, FAK-heterozygous ECs have an increase in both basal and serum-stimulated activation of Akt. Previous genetic studies have indicated a pro-angiogenic role for Akt [43] . More importantly, it has been reported that sustained activation of Akt in ECs resulted in enhanced blood vessel size and permeability and increased tumour growth [44] . Our findings, although correlative, suggest that the increased activity of Akt in FAK-heterozygous ECs could be responsible for the enhanced cellular proliferation and cause elevated angiogenic responses in the FAK-heterozygous mice. In the ex vivo aortic ring assay, a suboptimal dose of the Akt VIII inhibitor had a greater impact on the angiogenic responses of FAK-heterozygotes when compared with wild-types, suggesting increased sensitivity to Akt inhibition. A recent report demonstrated that FAK can bind Akt1 independently of the phosphorylation status of Y397 and that partial depletion of FAK, using short interfering RNA, stimulated basal phosphorylation of Akt [45] . Thus, we speculate that there may be a link between reduced FAK expression levels, a misbalance of FAK-phosphorylation and Akt activity that may enhance angiogenic responses. The mechanisms by which endothelial FAK levels control survival are not clear. It is tempting to speculate that as FAK has both kinase and non-kinase functions [46] , and the non-kinase-adaptor functions of FAK can regulate cellular proliferation via p53 without affecting cell migration [18] , [47] , that heterozygous FAK expression may bias for such scaffolding FAK functions. FAK can also regulate internalization of surface molecules and affect cell survival [48] . Thus, we postulate that signalling downstream of FAK, in FAK-heterozygous cells, regulates the expression or trafficking of pro-angiogenic cell surface markers, thereby affecting survival but not migration of these cells. Lastly, other studies have shown that loss of FAK expression or function can induce a change in Src-induced autophagy and thus enhance cell viability [49] . Although beyond the scope of this study it would be of interest to test these ideas in future experiments. The enhanced angiogenic affect of stromal FAK heterozygosity raises the possibility that low doses of FAK inhibitors may phenocopy the response in FAK-heterozygous mice. Our data indicate that this indeed may be the case as low doses of FAK inhibitor PF573228 enhanced microvessel sprouting ex vivo , although 0.01 μM PF573228 does not appear to affect autophosphorylation of FAK at Y397 in vitro (J.P., unpublished data). Furthermore, low doses of PF573228 increased tumour growth and angiogenesis. We have no evidence that such low doses prevail when such inhibitors are given at the maximal tolerated doses, where they have been shown to inhibit tumour growth and angiogenic effects [27] , [28] , [29] , or indeed how low doses may affect the tumour cells themselves. Off target effects of this inhibitor cannot be excluded or it is not shown if this applies to other FAK inhibitors. Instead, our results reveal new information about the basic biology behind the role of FAK in angiogenesis and provide proof-of-principle that reducing stromal-FAK either by genetic ablation or by pharmacological intervention can elevate angiogenic responses. This work highlights a novel function of FAK in the regulation of angiogenesis that depends on the levels of FAK expression, and not simply its presence. Primary cell cultures Primary mouse lung ECs were isolated and cultured as described previously [50] from either FAK-heterozygous or wild-type control mice. Tissue culture plates for all experiments were coated with a mixture of collagen (30 μg ml −1 ), gelatin (0.1%) and fibronectin (10 μg ml −1 ). In vivo tumour growth Age- and sex-matched FAK-heterozygous [20] and wild-type littermate controls on a mixed C57BL6/129 background were given a single subcutaneous injection into the flank of either 1 × 10 6 B16F0 melanoma cells, or 0.5 × 10 6 CMT19T lung carcinoma cells (ATCC). Tumour dimensions were measured everyday and the tumour growth was determined using the formula length × width 2 × 0.52. Fourteen days after injection or when tumour reached the maximum legal size allowed, mice were killed, tumour sizes measured and tumour samples were either snap-frozen or fixed in 4% paraformaldehyde for histological analysis. Immunohistochemical analysis Tumours were bisected and midline sections immunostained for endomucin or PECAM to detect blood vessels ECs and smooth muscle actin conjugated to Cy3 to detect smooth muscle cells as described [51] . Blood vessel density was calculated by counting the number of blood vessels per mm 2 of midline section. Smooth muscle cell coverage was determined by calculating the ratio of smooth muscle cell-positive blood vessels over total blood vessels [15] . Perfused blood vessels were detected by intravenously injection of Phycoerythrin-labelled PECAM antibody (100 μg) 15 min before B16F0 tumour excision. The percentage of perfused/functional blood vessels was calculated by the ratio of PE-PECAM-positive perfused vessels over the total blood vessels, detected by staining for endomucin across whole-tumour sections. As a control, transverse sections of unchallenged skin were also immunostained for endomucin or PECAM and blood vessel density was calculated by counting the number of blood vessels per mm 2 of skin dermis/section. To examine tumour ECs proliferation, mice received an intraperitoneal injection of 200 μl BrdU (5 mg ml −1 ) and 30 min later were killed and B16F0 tumours were dissected and processed for histological analysis. Double staining for endomucin and BrdU incorporation was carried out, and endothelial proliferation was calculated as the number of BrdU-positive cells per perimeter of blood vessels. Subcutaneous tumour-free angiogenesis assay Briefly, two autoclaved synthetic sponges (a kind gift from Daryl Harmon, Caligen Foam Ltd.) of ~1 cm 3 in size were implanted subcutaneously in the flanks of anaesthetized mice. Every 2 days, sponges were injected in situ with either 100 μl of PBS alone or 100 μl of PBS containing 10 ng ml −1 VEGF. After 14 days, sponges were excised and fixed for paraffin embedding. Sections of sponges were immunostained for vWF to identify blood vessels. Briefly, paraffin sections were dewaxed in xylene, hydrated by sequential immersion in 100, 80, 70 and 50% ethanol solutions and treated with protein kinase for 15 min at 37 °C. Sections were blocked with 2% normal goat serum, 1% BSA and 0.1% TritonX-100 and incubated with anti-vWF (AbD Serotec) overnight at 4 °C, followed by a Alexa-488-conjugated secondary antibody (Invitrogen) for 1 h at room temperature. Blood vessel density was assessed by counting the number of vWF-positive blood vessels per mm 2 of sponge section. The nuclear marker 4',6-diamidino-2-phenylindole was used as a counterstain. WST-1 assay Primary mouse lung ECs were seeded at a density of 2,500 cells per well in coated 96-well plates. EC medium was changed every 2 days. At each time point, 1 day, 2 days and 4 days, the cell proliferation reagent, WST-1 (Roche Applied Science) was applied to each well. Following 3 h incubation at 37 ° C, the absorbance of the samples was measured at 450 nm using an Anthos 2001 microplate reader. Wells without cells but containing complete medium and WST-1 acted as baseline absorbance controls. Results were normalized to data from day 1. Cell migration assay Primary ECs grown on glass coverslips were serum starved for 4 h in Opti-MEM. The coverslips were then placed ‘face-down’ onto Dunn chambers that contained Opti-MEM within the central chamber, and Opti-MEM with serum or VEGF in the outer chamber. Cells were then imaged at the ‘bridge’ between the two chambers, and tracked to determine speed and persistence of cellular movement. Two-dimensional tubulogenesis assay Primary mouse lung ECs were serum starved for 4 h in Opti-MEM. Cells were then detached from the plate and resuspended in Opti-MEM (supplemented with 1% fetal calf serum (FCS)). Fifty-thousand cells were seeded onto solid Matrigel (three wells per condition) in a 48-well plate. Images of the tubes were recorded using a phase contrast × 10 objective lens at 7 h after seeding. The area captured by the camera was considered the field of view and 3–4 complete fields per well were quantified. The total sum length of tube network per field was quantified. Three-dimensional EC sprouting assay Primary mouse lung ECs were incubated with a suspension of Cytodex glass beads (GE Healthcare) in EGM-2 medium (Lonza) at 37 ° C for 4 h with agitation every 20 min. This cell-bead suspension was then plated into flasks and left overnight. The following day, the coated beads were resuspended gently in 1 mg ml −1 fibrinogen solution (Invitrogen) with 0.15 units per ml of aprotinin solution (Invitrogen) and transferred to 24-well plates with each well containing a drop of thrombin solution (Invitrogen). Plates were left at room temperature for 15 min and then placed at 37 ° C for 1 h to allow the combined solution to clot. Finally, mitomycin-inactivated NIH-3T3 fibroblasts were then added to each well and allowed to settle for 3 h before changing the medium. Cells were fed with EGM-2 medium supplemented with 2% FCS with 30 ng ml −1 VEGF or PBS every 2 days and sprouts counted daily from day 3 to day 6. Immunofluorescence of cultured cells Cells grown on 10-mm glass coverslips were washed once in PBS, fixed in acetone for 5 min at −20 °C, washed in PBS three times and then blocked with 5% normal goat serum for 30 min at room temperature. After washing the cells once in PBS, cells were incubated with anti-FAK (1:100, BD-Biosciences cat. no 610087), anti-phospho-FAK (1:100, Invitrogen cat. no 44624, 44626) and anti-talin (1:100, Sigma T3287) antibodies for 1 h at room temperature. Alternatively, cells were washed once in PBS, fixed in 4% paraformaldehyde for 10 min, rinsed in PBS, permeabilized in 0.5% NP40 for 10 min and blocked with 0.1% BSA/0.2% Triton-X100 for 10 min before incubation with anti-paxillin (1:100 BD-Biosciences 610051), anti-vinculin (1:400 Sigma cat. no V9131) and Rhodamine-phalloidin for F-actin (1:1000 Invitrogen R415). Cells were then washed with PBS and incubated with Alexa-Fluor-conjugated secondary antibodies (1:100, Invitrogen) for 45 min at room temperature before being mounted on microscope slides using Prolong Gold anti-fade reagent (Invitrogen). Fluorescence microscopy was performed using a CCD (charge-coupled device) camera Hamamatsu C4742-95 and a Zeiss Axioplan microscope. Identical settings were used to acquire the images in both wild-type and FAK-heterozygous cells. The mean fluorescent intensity of total FAK, pY397-FAK and pY861-FAK in the whole-cell area was calculated using the ImageJ software. Western blot analysis For analysis of protein levels, cells were either lysed directly, or serum starved for 4 h and then serum-stimulated for 0, 5, 15, 30 and 60 min before lysis. Western blot analysis was performed as described in Supplementary Methods . The anti-, total FAK, pPyk2, total-Pyk2, p-Erk, total-Erk, pAkt (Ser473) and total Akt antibodies were from Cell Signaling Technologies (cat no. 3285, 3291, 3292, 9101, 9102, 9271 and 4685, respectively) The phospho-tyrosine FAK antibodies were from Invitrogen (cat. no. 44626, 44624). The anti-talin and anti-vinculin were from Sigma-Aldrich (cat no. T3287 and V9131, respectively). The anti-HSC70 and anti-paxillin were from Santa Cruz Biotechnology (cat. no. sc-24 and sc-5574). All primary antibodies were used in 1:1000 dilution in 3% BSA or 5% skimmed milk besides the anti-HSC70 and the anti-talin that were used in 1:5000 dilution and 1:500, respectively. Densitometric readings of band intensities were obtained using the ImageJ software. Ex vivo aortic ring assay with Akt inhibitor Thoracic aortas were isolated and prepared for culture as described previously [52] . Briefly, 1 mm thick rings were serum starved for 18 h at 37 °C before being embedded in growth factor-reduced Matrigel (BD-Biosciences) and cultured in medium supplemented with 2.5% FCS with or without Akt kinase inhibitor VIII (Calbiochem, Millipore), at concentrations indicated. Rings were fed every 2 days with fresh medium containing 2.5% FCS and the indicated concentration of the inhibitor. Sprouting microvessels were counted after 6 days. Ethical regulations All animal experiments were performed in accordance with UK Home Office regulations and the European Legal Framework for the Protection of animals used for scientific purposes (European Directive 86/609/EEC). Statistical analysis Statistical significance was calculated with unpaired Student’s t -test and P <0.05 was considered statistically significant, unless otherwise indicated. For tumour growth statistics, non-parametric Mann–Whitney U rank-sum test was performed to compare tumour volumes of each day. For Akt inhibition studies of aortic ring sprouting, data is presented using the log scale for the concentration of Akt inhibitor and statistical analysis between wild-type and FAK-heterozygous aortic rings at each concentration of Akt inhibitor was performed using multiple Student’s t -test and P <0.05 was considered statistically significant. How to cite this article: Kostourou, V. et al . FAK-heterozygous mice display enhanced tumour angiogenesis. Nat. Commun. 4:2020 doi: 10.1038/ncomms3020 (2013).